Titania single crystals with a curved surface Owing to its scientific and technological importance, crystallization as a ubiquitous phenomenon has been widely studied over centuries. Well-developed single crystals are generally enclosed by regular flat facets spontaneously to form polyhedral morphologies because of the well-known self-confinement principle for crystal growth. However, in nature, complex single crystalline calcitic skeleton of biological organisms generally has a curved external surface formed by specific interactions between organic moieties and biocompatible minerals. Here we show a new class of crystal surface of TiO 2 , which is enclosed by quasi continuous high-index microfacets and thus has a unique truncated biconic morphology. Such single crystals may open a new direction for crystal growth study since, in principle, crystal growth rates of all facets between two normal {101} and {011} crystal surfaces are almost identical. In other words, the facet with continuous Miller index can exist because of the continuous curvature on the crystal surface. Understanding the principles that determine crystal shape is a major challenge in many fields [1] , [2] , [3] , [4] , [5] , [6] , [7] , [8] . Theoretical studies of crystal morphology including Wulff construction and current models of crystal growth mechanisms are all underpinned by a consensus that crystals are convex polyhedrons and the interface between crystals and surrounding media is flat [1] . Such Wulff equilibrium crystal morphology has been extensively explored theoretically and experimentally for numerous atomic, molecular or even nanoparticle crystallization processes [9] , [10] , [11] , [12] . However, in nature, crystals with curved external surface, such as calcitic skeleton of biological organisms, usually exhibit unique mechanical property, light-management capacity and biological compatibility [13] , [14] , [15] , [16] . Unfortunately, continuous curved surface has been scarcely discovered in artificial single crystals. As an important semiconductor, TiO 2 crystals have attracted intense research interests owing to its potential applications in a wide range of fields such as catalysis, photovoltaic cells, photochromic devices and gas sensors [17] , [18] , [19] , [20] , [21] , [22] , [23] , [24] , [25] , [26] , [27] , [28] . For TiO 2 crystals in the anatase phase, the equilibrium shape built through Wulff construction is a slightly truncated tetragonal bipyramid enclosed by eight thermodynamically stable {101} facets and two {001} facets [29] , [30] , [31] . Here we demonstrate a facile synthetic strategy to prepare unconventional TiO 2 single crystals with a curved surface, in which organic citric acid (CA) and inorganic hydrofluoric acid (HF) were used as synergistic capping agents. Such curved surfaces of TiO 2 in anatase and rutile phase are composed of quasi continuous high-index microfacets. Moreover, we investigate the formation mechanism of curved crystal surface by density functional theory (DFT) calculations, which suggest the key role of synergistic effects of chemisorbed HF and CA and, particularly, the concentration of CA and its competitive adsorption on the high-index surfaces (such as (112)) that provide unique stabilization effect on the formation of bicone-like curved anatase TiO 2 . The synthetic strategy in this work may be applied to other functional crystals, with practical applications in catalysis, photonics and bio-inspired materials. Synthesis and characterizations of round anatase TiO 2 The synthetic approach used in this work was on the basis of the method of Yang et al . [19] via a hydrothermal reaction of titanium tetrafluoride (TiF 4 ), HF and CA as the precursor and co-capping agents, respectively. The inorganic capping agent of HF shows strong bonding to titanium species that could provide effective means for regulating the rate of hydrolysis and stabilizing specific high-reactive surfaces, such as (001) (refs 19 , 32 ). In the inset of Fig. 1a , we present the molecular structure of CA, which contains three carboxyl groups and one hydroxyl group; these molecular characteristics may provide various chemisorbed configurations on specific crystal surfaces, including monodentate, bidentate and/or other configurations [3] . 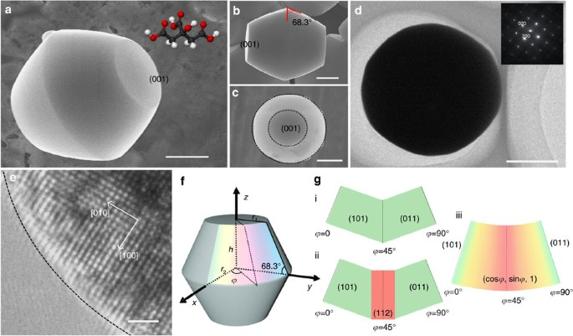Figure 1: Structural determination and geometric analysis of round anatase TiO2single crystals. (a–c) High-magnification SEM images of the as-prepared anatase TiO2single crystals viewed from various orientations. The inset inashows three-dimensional (3D) molecular structure of the organic capping agent (CA). (d) Typical TEM images of a round anatase TiO2single crystal indexed with [001] incidence. Single-crystal characteristic of anatase TiO2phase can be confirmed by the SAED pattern in the inset. (e) High-resolution TEM image taken fromcwith [001] orientation. (f) Schematic illustration of the geometric model of the round anatase TiO2single crystals.ϕ, Azimuthal angle in spherical coordinate system. (g) Unfolded views of the facets (presented by different colours) of crystals synthesized with CA concentrations of (i) 0, (ii) 0.127 M and (iii) 0.476 M. Scale bars are 1 μm ina–dand 1 nm ine. Figure 1: Structural determination and geometric analysis of round anatase TiO 2 single crystals. ( a – c ) High-magnification SEM images of the as-prepared anatase TiO 2 single crystals viewed from various orientations. The inset in a shows three-dimensional (3D) molecular structure of the organic capping agent (CA). ( d ) Typical TEM images of a round anatase TiO 2 single crystal indexed with [001] incidence. Single-crystal characteristic of anatase TiO 2 phase can be confirmed by the SAED pattern in the inset. ( e ) High-resolution TEM image taken from c with [001] orientation. ( f ) Schematic illustration of the geometric model of the round anatase TiO 2 single crystals. ϕ , Azimuthal angle in spherical coordinate system. ( g ) Unfolded views of the facets (presented by different colours) of crystals synthesized with CA concentrations of (i) 0, (ii) 0.127 M and (iii) 0.476 M. Scale bars are 1 μm in a – d and 1 nm in e . Full size image In contrast to the prior examples of faceted microcrystals [4] , [19] , the typical scanning electron microscope (SEM) images of the products reveal truncated biconic-shaped crystals with curved surface as shown in Fig. 1a–c . All diffraction peaks in the X-ray diffraction (XRD) pattern can be well indexed to the crystal structure of anatase TiO 2 phase (space group I 4 1 / amd , JCPDS No. 21-1,272) [33] , in good consistence with Raman data ( Supplementary Fig. 1 ). The single crystal characteristic of the products was further confirmed using transmission electron microscopy (TEM) and corresponding selected area electron diffraction (SAED) pattern, as shown in Fig. 1d . According to the crystallographic symmetries of anatase TiO 2 , the flat surfaces at both truncated ends must be {001} facets (further evidence is given in Fig. 1d ). The round crystal profile of curved surface ( Fig. 1d ) reveals that the crystals may be enclosed by quasi continuous microfacets, rather than flat surfaces, implying the equal growth rates of any facets other than {001}. High-resolution TEM image in Fig. 1e allows a direct view of the surface features of the curved microfacets. Evidently, the atomic arrangements of crystal surfaces change gradually resulting in quasi continuous vicinal microfacets, illustrating that our synthetic method favours a non-confinement growth by forming numerous high-index microfacets. We then statistically analysed the geometric characteristics with a schematic model ( Fig. 1f ) of an ideally round anatase TiO 2 single crystal. For the sample shown in Fig. 1a , the average radius of the fringe circle ( r 1 ), the middle circle ( r 2 ) and the height ( h ) are 1.14, 1.94 and 1.97 μm, respectively ( Supplementary Fig. 2 ). Further analysis based on these statistical results reveals that the interfacial angle between the frustum base plane and slant edge is 67.87° on average, being consistent with the interfacial angle between {001} and {101} facets of classical well-developed anatase TiO 2 single crystals [34] . Compared with the sample in Fig. 2 , the anatase crystals obtained in shorter reaction times are also enclosed by curved surfaces with a smaller size ( Supplementary Fig. 3 ). 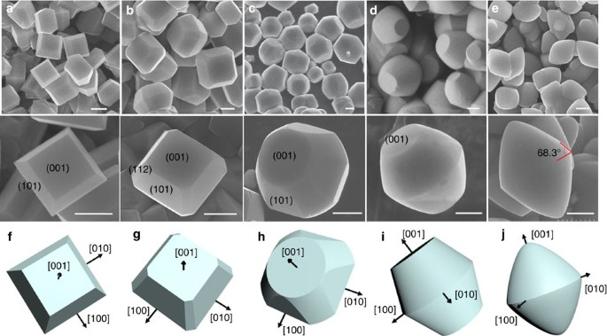Figure 2: SEM images and corresponding geometric models of anatase TiO2single crystals synthesized with different amounts of CA. (a) Truncated octahedral bipyramidal anatase TiO2single crystals with exposed {001} and {101} facets. (b) Polyhedral anatase TiO2single crystals exposed with {001}, {101} and {112} facets. (c) Polyhedral anatase TiO2single crystals enclosed with {001}, {101} and quasi continuous microfacets. (d) Round anatase TiO2single crystals exposed with {001} and quasi continuous microfacets. (e) Round anatase TiO2single crystals only exposed with quasi continuous microfacets. Scale bars are 1 μm. All crystals were synthesized in 5.33 mM TiF4aqueous solution with 0 g (a), 0.8 g (b), 1.5 g (c), 3 g (d) and 6 g (e) of CA at 180 °C for 20 h. Panelsf–jare corresponding geometric models shown ina–e. Figure 2: SEM images and corresponding geometric models of anatase TiO 2 single crystals synthesized with different amounts of CA. ( a ) Truncated octahedral bipyramidal anatase TiO 2 single crystals with exposed {001} and {101} facets. ( b ) Polyhedral anatase TiO 2 single crystals exposed with {001}, {101} and {112} facets. ( c ) Polyhedral anatase TiO 2 single crystals enclosed with {001}, {101} and quasi continuous microfacets. ( d ) Round anatase TiO 2 single crystals exposed with {001} and quasi continuous microfacets. ( e ) Round anatase TiO 2 single crystals only exposed with quasi continuous microfacets. Scale bars are 1 μm. All crystals were synthesized in 5.33 mM TiF 4 aqueous solution with 0 g ( a ), 0.8 g ( b ), 1.5 g ( c ), 3 g ( d ) and 6 g ( e ) of CA at 180 °C for 20 h. Panels f – j are corresponding geometric models shown in a – e . Full size image Regarding the important role of CA in the formation of curved anatase TiO 2 single crystal surfaces, we first investigated its concentration effect when the amount of fluorine was kept constant in these experiments. Without CA, only truncated bipyramidal-shaped TiO 2 single crystals ( Fig. 2a ) can be prepared through the anisotropic growth along {101} and {001} facets [19] . Interestingly, when 0.127 M CA·H 2 O was added into the reaction media, additional {112} facets first evolved along the crystal edges between the two {101} facets (see Fig. 2b ). For anatase TiO 2 single crystals synthesized with 0.238 M CA·H 2 O, more microfacets are exposed along the crystal edges and these quasi continuous microfacets clearly show some curvature at this stage ( Fig. 2c ). At 0.476 M CA·H 2 O ( Fig. 2d ), round anatase TiO 2 single crystal surfaces can be observed, suggesting the surface transformation from flat ones to quasi continuous high-index facets. Furthermore, by using 0.952 M CA·H 2 O, the obtained anatase TiO 2 crystals exhibit uniform bicone-like morphology without any flat surface as in the nonconfinement growth ( Fig. 2e ). It has been illustrated in Fig. 2d,e , that the interfacial angles between quasi continuous microfacets and {001} are always kept at 68.30°. Thus, the relative proportion of flat surfaces versus curved microfacets is largely dependent on the concentration of CA·H 2 O in the reaction mixture, which emphasized its unique effect of CA as an organic capping agent. To better describe this crystal-formation behaviour, we present the unfolded views of the crystal surfaces ( Fig. 1g ) in which all vicinal facets are shown in different colours. The varying varieties and size of the coloured surfaces reflect the continuous change of the external crystal facets that can be fulfilled by the addition of organic capping agents. As the concentrations of CA·H 2 O changed from 0 to a certain value, the facets of the unfolded parts for each individual crystals only correspond to two {101} facets at the beginning, and then give two {101} facets together with some minor {112} facets. The unfolded crystal facets finally evolve into countless small vicinal microfacets with continuously changing index. Combining the SEM and TEM results, we therefore refer to this synthetic method by using synergistic inorganic–organic capping agents as a non-confinement growth. Extending curved surface into rutile TiO 2 crystals The preferable adsorption of capping agents at specific facets is believed to determine the shape of the prepared nanoparticles [35] , [36] , [37] . Therefore, further insight into the functionality of the molecular structures of organic capping agents was obtained by systematically testing five other hydroxyl acids ( Fig. 3a–e ). The crystal characteristics were confirmed using XRD spectra, TEM images and the SAED patterns (see details in Supplementary Figs 4 and 5 ). Lactic acid (CH 3 CH(OH)COOH) and glycolic acid (CH 2 (OH)COOH) have similar structures as they both have one carboxyl and one hydroxyl group, although the former contains one more methyl group. Both these capping agents give rise to curved convex disk-shaped rutile crystals with four {111} facets, as illustrated in Fig. 3f,g . The difference in thickness of the rutile crystals might be attributed to the additional methyl group in lactic acid. When using malic acid (HOOCCH 2 CH(OH)COOH) with two carboxyl groups, octahedral rutile crystals were obtained with curved crystal edges ( Fig. 3h ). Interestingly, if we use tartaric acid (HOOCCH(OH)CH(OH)COOH) with even more hydroxyl groups, well-curved convex disk-shaped rutile crystals were prepared as shown in Fig. 3i . For the capping agents with more than two functional groups, new chemisorbed configurations may occur that favour the capping agents’ adsorption and further produce well-curved crystals without any flat surface. By contrast, the capping agent containing rigid benzene ring structures such as salicylic acid (C 6 H 4 (OH)COOH) can only lead to the formation of truncated bipyramidal TiO 2 anatase single crystals that can be rationalized by the reduced molecular flexibility and large steric hindrance of the benzene in backbone ( Fig. 3j ). Hence, the number of functional groups, molecular flexibility and steric hindrance may play a decisive role in the interaction of carboxyl and hydroxyl groups in the organic capping agents with crystal surfaces, which then results in substantial difference in morphologies and crystallographic polymorphs of TiO 2 . 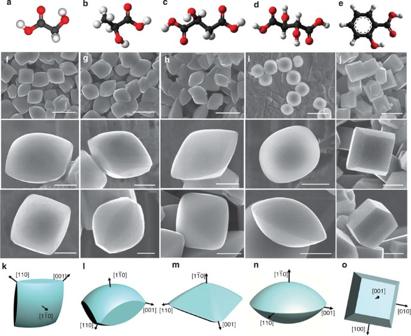Figure 3: Controlling morphology and polymorph of round TiO2single crystals via molecular structures of organic acids. (a–e) 3D molecular structures of glycolic acid, lactic acid, malic acid, tartaric acid and salicylic acid as the organic capping agents. (f–j) SEM images and (k–o), corresponding geometric models of rutile TiO2single crystals synthesized with the organic acids as shown ina–e. Scale bars of the images in first line and others are 5 and 1 μm, respectively. Note: anatase TiO2single crystals were obtained by using salicylic acid. Figure 3: Controlling morphology and polymorph of round TiO 2 single crystals via molecular structures of organic acids. ( a – e ) 3D molecular structures of glycolic acid, lactic acid, malic acid, tartaric acid and salicylic acid as the organic capping agents. ( f – j ) SEM images and ( k – o ), corresponding geometric models of rutile TiO 2 single crystals synthesized with the organic acids as shown in a – e . Scale bars of the images in first line and others are 5 and 1 μm, respectively. Note: anatase TiO 2 single crystals were obtained by using salicylic acid. Full size image Synergistic effect of organic–inorganic capping agents Moreover, no well-faceted anatase TiO 2 single crystals can be synthesized in the absence of HF and CA as reported previously [19] , and the surfaces of these crystals are flat with small square shape that is likely to be (001) facets of anatase TiO 2 ( Supplementary Figs 2 and 6 ). Without hydrofluoric acid, only spherical polycrystalline anatase TiO 2 particles were prepared with irregular surfaces and, more importantly, no {112} facets and well-curved crystals can be observed even at high CA concentration. We therefore further believe that the essential factor for the nonconfinement growth is the synergistic effect of hydrofluoric and hydroxyl acids. In order to better understand these experimental observations, we then performed systematic DFT calculations to illuminate the energetic origins of the synergistic effects of the different capping agents. Anatase TiO 2 surfaces were modelled by periodic slabs, and 1 × 2 and 2 × 2 surface cells were used for (101) and (112) surfaces, respectively. For the anatase TiO 2 (112) surface, two different termination structures were considered in this work. The bulk-truncated (112) surface exhibits small dentate conformation, with unsaturated O 2c and Ti 5c being exposed ( Supplementary Fig. 7 ). Interestingly, we also found that by removing half of the dentate structural units from each surface cell we can actually obtain the 2 × 1 reconstructed (112) surface (see Supplementary Fig. 7 ). Such termination with bigger dentate and much less compact conformation can undergo drastic relaxation during optimization. Accordingly, these two surfaces, donated as (112)-s and (112)-b, give the calculated surface energies of 0.73 and 0.65 J m −2 , respectively. To study the interaction between capping agents and crystal surfaces, we considered various possible configurations for the adsorption of HF and CA at (101), (112)-s and (112)-b surfaces. For their single adsorption, at most 8 (1), 16 (4) and 16 (1) HF (CA) molecules can adsorb at slab surfaces (top and bottom) of the (101), (112)-s and (112)-b slabs, respectively. The dissociative adsorption of HF gives rise to the formation of surface hydroxyls as well as Ti–F species and, for CA, each molecule forms two O–Ti bonds at the (112)-s and (112)-b surfaces but only one O–Ti bond at (101) ( Supplementary Fig. 8 ). However, it should be noted that the dissociated CA at anatase TiO 2 (112)-s forms the two O–Ti bonds at one carboxyl group in bidentate configuration, while that at (112)-b forms the two O–Ti bonds at two carboxyl groups each and the CA adsorbs molecularly intact at (101). The adsorption energies of HF and CA molecules were calculated by taking into consideration the solvation effect, and the results are listed in Supplementary Table 1, 2 and Table 1 (see equation 2). As we can see from the calculated average adsorption energies ( Table 1 ), the bonding strengths of HF at the various (101) and (112) surfaces are very similar. However, for CA, it gives much higher adsorption energy (3.07 eV) at (112)-b than that at (101) (1.02 eV) or the other (112) surface (0.51 eV). This could be simply because that the adsorption configurations for dissociated HF at all the surfaces are very similar, while those for CA are quite different and only the dissociated CA at the (112)-b surface can form two strong O–Ti bonds and multiple H bonds between the three carboxyl groups and surface O. These results clearly indicate that the coexistence of CA in capping agents would have strong tendency to favour the occurrence of (112)-b surfaces. Moreover, considering that the extraordinarily strong interaction between CA and (112)-b occurs at the characteristic V-type ‘ditch’ structure, one may also expect that, with the increasing amount of CA in the synergistic capping agents, (112)-b facets would occur first since it has the highest concentration of such ‘ditch’ structure and other high-index vicinal surfaces containing both (101) terrace and (112)-b would then gradually form. In addition, the preferential adsorption at surface ‘ditch’ structures may largely explain why other polyacid or flexible hydroxyl acid agents can have similar synergistic capping effect as CA as we have determined in our experimental studies. In fact, by carefully analysing the SEM images of the rutile crystals prepared in this work, we can find that the curved surfaces are initiated at the facets, which also gives clear ‘ditch’ structure (see Supplementary Fig. 9 ). Table 1 Calculated average adsorption energies of HF and CA at TiO 2 (101), (112)-s and (112)-b surfaces in solution. Full size table To further verify the synergistic effect of capping agents on the TiO 2 morphologies, we also made Wulff construction plots ( Fig. 4 ) by using the surface energies ( Table 2 ) estimated by taking into consideration the adsorption and solvation effect of capping agents. It should be noted that, as one can see from Supplementary Fig. 8d,f , the favourable adsorption of the CA molecule at (101) and (112)-b surfaces still leaves free Ti 5c and O 2c sites because of its big size. Therefore, considering the coexistence of the two capping agents in solution, we calculated the surfaces with all the free sites occupied by dissociated HF. As shown in Fig. 4 , the TiO 2 crystal covered by CA and HF gives rise to the shape in line with the experimental observation in the current work (see Fig. 2c ), again confirming that such carboxylic acids can work as the co-capping agents with HF to favour the formation of the high-index surfaces and the corresponding biconic-shaped crystals with quasi continuous microfacets. 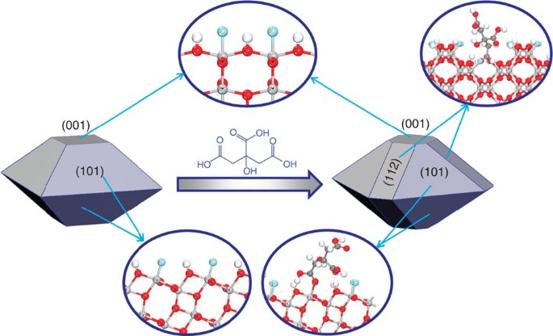Figure 4: HF and CA molecules chemisorbed on TiO2crystal surfaces. The polyhedrons are 3D Wulff construction diagrams of the anatase TiO2crystals using the surface energies of HF-covered (001)/(101) (left), and CA/HF-covered (101) and (112)-b facets (right) in solution. The insets show the atomic model of capping agents (co-)chemisorbed on different crystal surfaces of anatase TiO2. Ti, O, H, F and C atoms are represented by balls in light grey, red, white, light blue and dark grey, respectively. Figure 4: HF and CA molecules chemisorbed on TiO 2 crystal surfaces. The polyhedrons are 3D Wulff construction diagrams of the anatase TiO 2 crystals using the surface energies of HF-covered (001)/(101) (left), and CA/HF-covered (101) and (112)-b facets (right) in solution. The insets show the atomic model of capping agents (co-)chemisorbed on different crystal surfaces of anatase TiO 2 . Ti, O, H, F and C atoms are represented by balls in light grey, red, white, light blue and dark grey, respectively. Full size image Table 2 Calculated surface energies (in J m −2 ) of the clean ( γ ) and HF/CA co-covered anatase TiO 2 (101) and (112)-b surfaces in solution ( γ ′). Full size table Using synergistic organic–inorganic capping agents, we successfully prepared titania single crystals with a thermodynamically unexpected shape. The surface of TiO 2 with regular curvature is composed of quasi continuous high-index microfacets and the Miller index (cos ϕ , sin ϕ , 1) of these microfacets also changes gradually between (101) and (011) crystal facets (see Supplementary Note 1 ). These findings cannot be readily understood with the classical anisotropic crystal growth theories such as crystal self-confinement and Wullf construction. Through DFT calculations, we found that the continuous bending of the external crystal surface can be attributed to the synergistic effects of chemisorbed hydrofluoric acid and CA and, particularly, the unique adsorption mode of organic CA that favours its attachment to high-index facets. We have also demonstrated the promise held by round TiO 2 single crystals both in anatase and rutile phases (shown in Figs 1 and 3d ) for the application as photocatalysts, with truncated bipyramidal-shaped anatase TiO 2 single crystals (faceted TiO 2 , shown in Fig. 2a ) as comparison. After removal of the capping agents, all the round TiO 2 crystals show higher photocatalytic activities than faceted TiO 2 crystals (see Supplementary Table 3 , Supplementary Figs 10 and 11 ). Moreover, this synthetic strategy provides the principles for designing a new family of functional crystals with a non-flat surface, which have potential applications in catalysis, photonics, bio-inspired materials and chemical–mechanical planarization of advanced integrated circuits and may also shed light on fundamental mechanisms of the organic–inorganic interactions in the biomineralization process. Synthesis of round TiO 2 single crystals Curved anatase TiO 2 crystals were synthesized by a modified procedure reported in ref. 19 . An aqueous TiF 4 (Aldrich Chemical) solution (5.33 mM) was prepared by dissolving TiF 4 in a weakly acidic solution that was adjusted to the pH of deionized water (~2.1) by the addition of hydrochloric acid (1.5 M). In a typical synthesis, 30 ml of TiF 4 aqueous solution was added into a 50-ml Teflon-lined reactor. Then 1.5 g CA monohydrate (C 6 H 8 O 7 ·H 2 O, Aldrich Chemical) was put into the reactor subsequently and the mixture was stirred for 5 min to form an aqueous solution by using a Teflon-coated magnetic stirrer bar. After that, 0.4 ml of hydrofluoric acid (10 wt%) was added to the above solution and the reactor was transferred into a stainless steel autoclave immediately. The Teflon-lined autoclave was kept at 180 °C for 14–24 h in an electric oven. The autoclave was then cooled to room temperature under ambient environment. The solid products were collected from the bottom of the vessel. After that, the curved anatase TiO 2 crystals were washed with deionized water three times and then dried in vacuum overnight. Material characterizations Crystallographic information of TiO 2 single crystals was obtained with XRD (Bruker D8 Advanced Diffractometer with Cu Kα radiation). The morphology and structure of the samples were characterized by high-resolution TEM and SAED (JEOL JEM-2010F) and field emission SEM (HITACHI S4800 and SEM, JOEL JSM 6380). Moreover, the crystal structure of the samples was determined with Raman spectroscopy (Renishaw, inVia+Reflex). Theoretical calculations DFT calculations have been performed with the PWScf code, which is part of the Quantum-Espresso package [38] . The plane-wave basis sets cutoffs for the smooth part of the wavefunctions and the augumented densities were 25 and 200 Ry, respectively. Electron–ion interactions were described using ultrasoft pseudopotentials [39] , with electrons from C, O, F 2 s , 2 p and Ti 3 s , 3 p , 3 d , 4 s shells were explicitly included in the calculations. For the anatase TiO 2 (101) and (112) surfaces, they were modelled by slabs with 4 and 9 layers, respectively, and corresponding 1 × 2 × 1 and 1 × 1 × 1 k-point meshes were used. The adsorption of HF and CA was modelled on both sides of the slab and, during optimization, all the slab and adsorbate atoms were allowed to move (force threshold was 0.05 eV Å −1 ). The surface energy of a clean anatase TiO 2 (101) surface was taken from an early DFT study in ref. 40 , which employed nearly the same set of calculation setting and code. The surface energies of clean (112) surfaces were calculated by using the following equation: where E slab is the total energy of the slab, is the energy of a bulk TiO 2 unit, n is the number of TiO 2 units in the slab and A is the exposed area of one side of the slab (the two sides of the slab are equivalent). Considering the solvation effect, we calculated the adsorption energies of HF and CA at the anatase TiO 2 surfaces by using the following equation: in which E surf is the total energy of the TiO 2 slab, E mol is the total energy of the adsorbed molecule (HF or CA) in the gas phase, E surf+mol is the total energy of the system with adsorbed molecules at the surface, E ad–sol and E mol–sol are the solvation energies of the HF (or CA)-covered slabs and a single HF or CA molecule, respectively. Specifically, calculations for E mol–sol were performed employing the Gaussian 03 computational software package [41] . PBEPBE correlation functional in combination with the 6–311++G (d,p) basis set were used [42] , [43] . The polarizable continuum model was employed to include solvent (H 2 O) effects. In order to estimate E ad–sol , we used the SIESTA code and the surface structures directly obtained from PWScf calculations [44] . The long-range electrostatic solvation effect for the systems in aqueous surroundings was taken into account by using a periodic continuum solvation model based on the modified Poisson–Boltzmann equation [45] , [46] , [47] . Moreover, in order to estimate the surface energies of surfaces covered by different capping agents in solution, the same strategy reported in a previous work was also used [48] . How to cite this article : Yang, S. et al . Titania single crystals with a curved surface. Nat. Commun. 5:5355 doi: 10.1038/ncomms6355 (2014).